Macroscopically local correlations can violate information causality Although quantum mechanics is a very successful theory, its foundations are still a subject of intense debate. One of the main problems is that quantum mechanics is based on abstract mathematical axioms, rather than on physical principles. Quantum information theory has recently provided new ideas from which one could obtain physical axioms constraining the resulting statistics one can obtain in experiments. Information causality (IC) and macroscopic locality (ML) are two principles recently proposed to solve this problem. However, none of them were proven to define the set of correlations one can observe. In this study, we show an extension of IC and study its consequences. It is shown that the two above-mentioned principles are inequivalent: if the correlations allowed by nature were the ones satisfying ML, IC would be violated. This gives more confidence in IC as a physical principle, defining the possible correlation allowed by nature. Despite quantum theory being almost a century old, its axioms remain mathematical in nature, and we are still searching for physical principles from which to derive it. After the initial discussions of the founding fathers, the operationalist viewpoint prevailed, and most were satisfied with a useful and strikingly precise theory. With the advent of quantum information science, however, a new source from which to draw principles of a more intuitive flavour was unveiled. Following this direction, many recent works have been devoted to study which tasks would be possible if correlations more general than the ones allowed by quantum mechanics could be achieved [1] , [2] , [3] , [4] , [5] , [6] , [7] , [8] . There are several motivations for these studies. First, they allow us to understand what is special about quantum mechanics, and consequently to get more intuition on it. Following this direction, results such as the impossibility of instantaneous transmission of information [1] and of cloning, the existence of monogamy of correlation, and secrecy [2] were shown not to be particular features of quantum mechanics. Second, if one finds a practical task limiting the correlations to be quantum, this would immediately gain the status of a physically motivated defining property of quantum correlations. Along these lines, constraints on distributed computing [3] , communication complexity [4] , [5] and the like can be thought of as candidate requisites from which the theory could in principle be derived. Finally, it could be possible that quantum mechanics is not the definitive description of nature, and more general correlations might be observed in the future. Thus, some physically motivated sets of correlations that are known to be bigger than the set of quantum correlations appear as candidates for possible generalizations of quantum mechanics. A pioneering effort in this direction was that of Popescu and Rohrlich [1] , who investigated whether the impossibility of transmitting information instantaneously (that is, the no-signalling principle) is enough to characterize the set of quantum correlations. It turned out that this was not the case. There exist sets of correlations satisfying the no-signalling principle that are not achievable in quantum physics. The tantamount example of this is given by the Popescu–Rohrlich (PR) box [1] . In this vein, other principles based on information-theoretic ideas were proposed as candidates from which the set of physically realizable correlations could be constrained [6] , [7] , [8] . In this work, we study two recent proposals: macroscopic locality (ML) [6] and information causality (IC) [7] . In a nutshell, ML states that the coarse-grained statistics of correlation experiments should admit a local hidden variable model, that is, those statistics that do not violate any Bell inequality [9] . IC, on the other hand, states that if Bob receives m bits of information from Alice, he cannot obtain more information about Alice's system than m bits, even if he shared with her some previous resource. For the m= 0 case, IC simply reduces to the no-signalling principle. Formally, IC is derived by introducing a game in which Bob has to guess one of Alice's independent and random bits (chosen at random), and bounding the sum of mutual information of Bob's different guesses with Alice's actual data by the amount of one-way communication from Alice to Bob. The purpose of this work is twofold. First, we extend the IC game to the case in which Alice's data are composed of d -dimensional alphabets ( dits ), of which Bob has to randomly guess one, allowing in principle for m dits of communication from Alice to Bob. As in the original case, we find an extremal non-signalling box that perfectly solves this task, and analyse the effect of adding noise to this set of correlations. The scenario we find in this case proves richer than the original, which allows us in turn to, second, show the inequivalence between IC and ML. In particular, we show that there exist correlations that satisfy ML, but violate IC. This implies that it is very unlikely that ML is the defining property of possibly obtainable correlations, as in this case one would have to accept that IC is violated. In this study, we start by reviewing the principle of ML, together with another attempt to characterize the quantum set of correlations: the Semi Definite Program (SDP) hierarchy by Navascués, Pironio and Acín (NPA) [10] , [11] , which is intimately related to the former. We then discuss the principle of IC by introducing our task, which generalizes the original one. We then analyse the newly found scenario and compare it with the previously known case, discussing the implications. It will be seen that, in the new scenarios studied here, IC comes closer to the quantum set than ML. This fact establishes IC as a more suitable candidate for a physical axiom defining the set of quantum correlations. Macroscopic locality and the NPA hierarchy Macroscopic locality [6] was introduced more as a principle producing an alternative to quantum theory than as an axiom for it. Since its inception, it was known that, when considered together with the no-signalling principle, it does not give rise to the set of quantum correlations, but, instead, to a larger set. This set is precisely the one labelled by Q 1 in refs [10] , [11] , that is, the first step in a hierarchy of SDPs that assymptotically converge to the quantum set. It was known already that, in some scenarios, further steps in the hierarchy are strictly contained in Q 1 , while also containing the quantum set [10] , [11] . Thus, it sufficed to prove the equivalence of Q 1 and the ML set to realize that this axiom would not suffice to fully determine quantum correlations. ML retains its interest, though, both as an example of a principle with physical content that can be put forth as a candidate for an axiom, and as a testable requirement from which a theory larger than quantum arises, and which could in principle be used to disprove quantum physics. As we mentioned before, it demands that classical physics be recovered in the large particle number limit by imposing that the coarse-grained correlations arising in an experiment involving a macroscopic number of particles can be modelled with local hidden variables. This requirement applied to microscopic probabilities is what gives Bell-local sets of correlations, which satisfy Bell inequalities. Less restraining, ML imposes this constraint on their macroscopic counterpart; all Bell-local correlations thus satisfy ML, but the converse fails to hold. To date, ML had not been contrasted with other attempts at axiomatizing quantum correlations from physical postulates. Information causality and its extension As we stated before, IC was introduced through the use of a game with two players, Alice and Bob, in which Alice is given N independent and unbiased bits of which Bob has to guess one, chosen at random. To achieve this, they can share before the game any amount of physical resources that they want (classical correlations, entangled states or, in a hypothetical scenario, non-local postquantum boxes), and Alice is further allowed to send m bits to Bob after she receives her input. We generalize this task by extending the alphabet size in which Alice's inputs range from 2 to an arbitrary number d . Bob then has to guess, again using previously shared resources but now allowing Alice to send him m dits , one of Alice's inputs, again chosen at random. IC, in fact, imposes a bound on where x K are Alice's independent and random input dits, y is Bob's random input telling him which x K to aim for and G is Bob's guess at that chunk of Alice's data. I ( x K : G|y = K ) is in turn the Shannon mutual information between Bob's guess and Alice's input x K , given that he aims at guessing that particular input. IC, stated in general, imposes that Although all quantum correlations satisfy this requirement, it is still an open question whether there are postquantum correlations that satisfy IC (ref. 12 ). We now study to what extent the IC condition defines the quantum set. To do this, we first consider a protocol that is independent of the resources shared by Alice and Bob. As will be seen, this protocol naturally suggests a non-signalling box as an optimal resource. We approach the quantum set by adding noise to this box and then ask how robust the IC violation is. We start by considering the case N =2. Alice and Bob share a box with d inputs on Alice's side and two inputs on Bob's, and d outputs on both sides ( Fig. 1 ). We label by a ( b ) the output of the box on Alice's (Bob's) side. The message Alice sends to Bob is M =( a–x 0 ) mod d , and Bob's guess is G =( b–M ) mod d =( b–a+x 0 ) mod d . 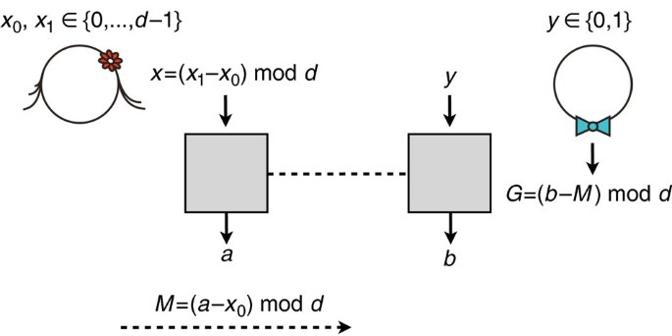Figure 1: Information causality protocol ford-dimensional alphabets. Suppose Alice (left) is given two dits,x0andx1, whereas Bob (right) gets a bity. Bob is asked to guess the value of one of Alice's dits, according to the value ofy. If Alice and Bob share the noiseless box 11 they can solve this problem perfectly. To do so, Alice inputs (x1–x0) moddinto the box, whereas Bob inputsy. After receiving her outputa, Alice sends a messageM=(a–x0) modd, corresponding to one dit of communication. Bob, in possession ofM, makes his guessG=(b–M) modd=(b–a+x0) mod d. Given that the box behaves asx.y=(b–a) modd, Bob computes the valueG=[(x1–x0).y+x0] modd, which equalsx0ify=0 andx1ify=1. Figure 1: Information causality protocol for d -dimensional alphabets. Suppose Alice (left) is given two dits, x 0 and x 1 , whereas Bob (right) gets a bit y . Bob is asked to guess the value of one of Alice's dits, according to the value of y . If Alice and Bob share the noiseless box 11 they can solve this problem perfectly. To do so, Alice inputs ( x 1 – x 0 ) mod d into the box, whereas Bob inputs y . After receiving her output a , Alice sends a message M =( a – x 0 ) mod d , corresponding to one dit of communication. Bob, in possession of M , makes his guess G= ( b–M ) mod d =( b–a + x 0 ) mod d. Given that the box behaves as x.y =( b–a ) mod d , Bob computes the value G =[( x 1 – x 0 ). y + x 0 ] mod d , which equals x 0 if y =0 and x 1 if y =1. Full size image The probability of Bob making a correct guess is where both Alice and Bob's inputs were unbiased. In the case y =0, the condition for a correct guess G = x 0 is equivalent to b–a =0 mod d . When y =1, we need to split the cases according to x=j with j =0, ..., d –1, and the correct guess condition G = x j is equivalent, in each case, to b–a = j mod d . Putting this together, we have for the success probability This expression says that if Alice and Bob share a box satisfying P ( x.y = ( b–a )mod d | xy) =1, this would lead to a probability of success equal to unity. This in turn would imply I =2 log 2 d , which violates the IC condition (2) as m =1. Such a box can be operationally defined as with a , b , x ∈ {0, ..., d –1}, and y ∈ {0, 1}. This is a generalization of the PR box [1] , to which it reduces in the case d =2. It is extremal in the d 2 dd non-signalling polytope (in this notation the first two numbers refer to Alice and Bob's input sizes, and the last numbers to their respective output sizes), as can be verified by using the same counting argument as in the proof of theorem 1 of ref. 14 . We now define an isotropic noisy box as follows: that is, a mixture of the generalized PR box (11) and box , representing classical random noise. Box outputs completely random dits, regardless of the inputs, and can be decomposed, as we did in the second line of equation (6), in terms of PR 0 plus d –1 other extremal non-signalling boxes, denoted by PR j with j ∈ {1, … , d –1}, s.t. The parameter E (0≤ E ≤1) quantifies the amount of noise in the box. These noisy correlations satisfy P ( B − A = x.y mod d | xy ) = (( d − 1) E + 1) / d hence we have for the success probability P S = (( d − 1) E + 1) / d . Although we could search for the critical value of E for a single box to stop violating IC, it was seen already in the original d =2 case that this is not optimal [7] . Instead, one needs to consider the task illustrated in Figure 1 for an arbitrary input size N , and extend the protocol described by nesting many instances of it. For the case of isotropic noisy boxes and d =2, it was seen that a suitable nesting of the protocol was enough to recover the quantum bound [7] . In the Methods section (see also Fig. 4), we describe this nesting and its extension to arbitrary dimension d . This extension proves straightforward, apart from the consideration of the cancellation of errors of different boxes, which now happens less frequently because of the larger outcome alphabet. We find a recurrence relation for the probability of success, and, by solving it, we obtain for the success probability of n boxes (see Methods) This is the probability of Bob producing a correct guess after the use of n boxes. Note that, given the structure of the nesting, one needs to use n =log 2 N boxes if the input consists of N dits. To study the violation of IC in terms of the probability of a successful guess, we use Fano's inequality [13] to bound I , as was already discussed for arbitrary d -dimensional alphabets in ref. 7 where h ( p )=− p log 2 p− (1− p )log 2 (1– p ) is the binary entropy, and we set equal probabilities for the correct guessing of the different dits, as is the case in the protocol. Considering this bound for success probability in the nested protocol given in equation (8), we obtain Consequences of the IC extension and inequivalence with ML We now turn to the consequences of the extension of IC that we have introduced. 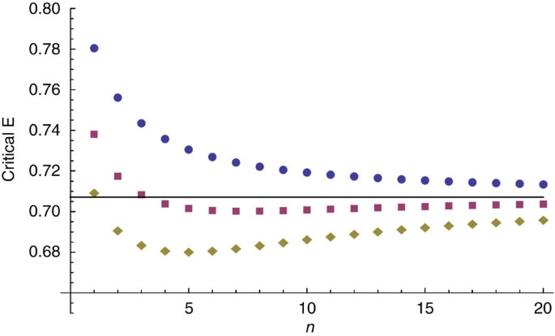Figure 2: Critical noise level for IC violation. We plot the critical amount of noise for which IC ceases to be violated, as a function ofn, and for different values ofd(d=2 circles,d=5 squares,d=10 diamonds). The solid line corresponds to, which, according to our numerical calculations up tod=5, coincides with ML. In Figure 2 we show the critical value of E for which IC ceases to be violated, as a function of the number of boxes used, n , and for different values of d . This value is obtained from (10). For d =2, the critical value of E asymptotically approaches Tsirelson's bound , which defines the extent of the quantum set for isotropic correlations. Therefore, we recover the result that IC defines isotropic quantum correlations for d =2, which also coincide with those satisfying ML (or, equivalently, are in Q 1 ). It was shown, however, that this protocol does not define the entire quantum boundary even for d =2 (ref. 12 ). Figure 2: Critical noise level for IC violation. We plot the critical amount of noise for which IC ceases to be violated, as a function of n , and for different values of d ( d =2 circles, d =5 squares, d =10 diamonds). The solid line corresponds to , which, according to our numerical calculations up to d =5, coincides with ML. Full size image For larger values of d , however, the situation proves richer. First, we notice that for sufficiently large d , the curves go below the critical value E T . This value is therefore no longer representative of the extent of quantum correlations. However, it still defines the extent of macroscopically local isotropic correlations, as we have checked for values of d up to 5 by solving the SDP that defines the set Q 1 . This thus proves the inequivalence of ML and IC. Table 1 summarizes the critical values obtained for the different sets. Table 1 Critical values of noise for increasing alphabet dimension. Full size table Unfortunately, contrary to the d =2 case, we do not know whether the amount of noise for which IC stops being violated coincides with the quantum boundary. The best bounds we know are the ones depicted in Table 1 . 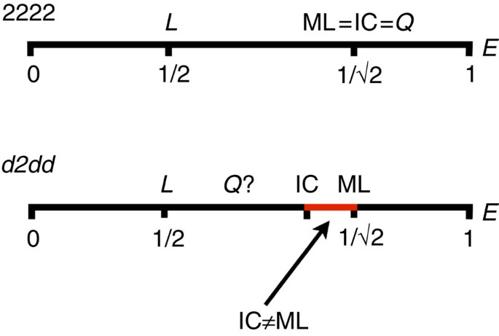Figure 3: Scenario comparison for the 2222 andd2ddcases. In the 2222 case, the amount of noiseE(see Equation (6)) for which IC and ML stop being violated coincides and equals. For the cased2ddwithd>2, the violation of IC can stand more noise than that of ML, which shows that ML correlations can violate IC. Note thatE=1 corresponds to no noise. We also depict the amount of noise for which the isotropic correlations have a classical local (L) and a quantum (Q) description. We sketch the situation pictorially in Figure 3 , where we compare the d =2 and larger d cases. Figure 3: Scenario comparison for the 2222 and d 2 dd cases. In the 2222 case, the amount of noise E (see Equation (6)) for which IC and ML stop being violated coincides and equals . For the case d 2 dd with d >2, the violation of IC can stand more noise than that of ML, which shows that ML correlations can violate IC. Note that E =1 corresponds to no noise. We also depict the amount of noise for which the isotropic correlations have a classical local ( L ) and a quantum ( Q ) description. Full size image The search for physical principles that could constrain the possible correlations observed in nature is still ongoing. The main goal of the present work was to develop one of these principles, IC, and compare it with another, ML. We formulated IC for arbitrary dimensions of the input alphabet and showed that IC imposes stronger constraints than ML on a family of correlations (the isotropic ones). These results put IC as a stronger candidate for a principle behind the correlations allowed by nature. The case for IC as the axiom defining quantum mechanics is reinforced. On the technical side, a curious feature appears in the curves presented in Figure 2 . In contrast to the d =2 case, in which the critical level of noise monotonously approaches E T , for larger values of d , the curves display a minimum in the critical noise for a finite value of n . The position of this minimum further decreases with increasing d . Although this effect is not yet fully understood, it might hint towards the non-optimality of the protocol considered. We leave this question for further investigations. As a final remark, we note that the extension remains valid in the d→∞ case. Interestingly, through this extension, Bob would be able to guess (to arbitrary precision) either one of two arbitrary precision floating point numbers of Alice using just one of the extremal d 2 dd boxes that we introduced. How this compares as a resource to an asymptotic number of standard PR 2222 boxes is a question for further study. Nesting the IC protocol In this study, we discuss the nesting of the protocol described in the main text needed to tackle the task when N >2. The nesting process is similar to that originally presented in ref. 7 , but differs in the treatment of accumulated errors. For clarity, suppose Alice is given N =4 dits, x 0 , x 1 , x 2 and x 3 , of which Bob has to learn one, indexed by the random bits he receives, y 0 and y 1 ( Fig. 4 ). Now Alice and Bob share three boxes. If these were the noiseless PR 0 boxes with a,b,x ∈ {0 , ..., d –1}, and y ∈ {0,1}, they could perfectly solve the task. The main idea (explained in detail in Fig. 4 ) is that they can use the first box to reveal the value of either x 0 or x 1 , and the second box to x 2 or x 3 . In the first case, Bob would have to know a message, M′ , whereas in the second he would have to know M ′′. As only one message can be transmitted, they use the third box to reveal to Bob either M ′ or M ′′, depending on which dit he wants to know. 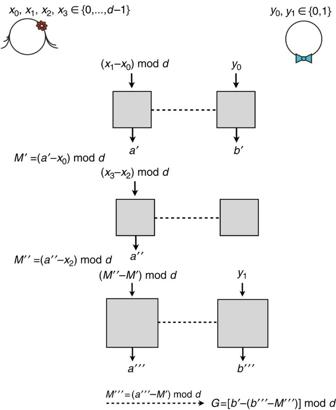Figure 4: Nesting of the protocol forN>2. We illustrate how to recursively use theN=2 protocol to solve the IC task for larger values ofN. Depicted is the case ofN=4, where Bob (right) aims to know the value of either of the four ditsx0,x1,x2orx3. Alice (left) inputs (x1–x0)moddin the first box, and would have to send the messageM′=(a′–x0)moddto enable Bob to know eitherx0orx1. She proceeds similarly in the second box, but now usingx2andx3. In this case, the message she would send would beM′′=(a′′–x2) modd. As she can send only one message, they use a third box to enable Bob to know eitherM′ orM′′. To this end, Alice inputs (M′′–M′) moddto the third box, and sends the messageM′′′=(M′′–M′) moddto Bob. By inputingy1=0,1 to the third Box, he can guess the value ofM′ orM′′, depending on which dit he is looking for. Having this information, he uses either box 1 or box 2 to discover the dit he aims for. In the figure, we supposed that Bob wants to know the value of eitherx0orx1. In this case, he would inputy1=0 into the third box, find the value ofM′, inputy0into the first box and finally guess the value of the bit he wants according toG=[b′–(b′′′–M′′′)] modd. For arbitraryN, this process can be iterated in a straightforward manner. Figure 4: Nesting of the protocol for N >2. We illustrate how to recursively use the N =2 protocol to solve the IC task for larger values of N . Depicted is the case of N =4, where Bob (right) aims to know the value of either of the four dits x 0 , x 1 , x 2 or x 3 . Alice (left) inputs ( x 1 – x 0 )mod d in the first box, and would have to send the message M ′=( a ′– x 0 )mod d to enable Bob to know either x 0 or x 1 . She proceeds similarly in the second box, but now using x 2 and x 3 . In this case, the message she would send would be M ′′=( a ′′– x 2 ) mod d . As she can send only one message, they use a third box to enable Bob to know either M ′ or M ′′. To this end, Alice inputs ( M ′′– M ′) mod d to the third box, and sends the message M ′′′=( M ′′– M ′) mod d to Bob. By inputing y 1 =0,1 to the third Box, he can guess the value of M ′ or M ′′, depending on which dit he is looking for. Having this information, he uses either box 1 or box 2 to discover the dit he aims for. In the figure, we supposed that Bob wants to know the value of either x 0 or x 1 . In this case, he would input y 1 =0 into the third box, find the value of M ′, input y 0 into the first box and finally guess the value of the bit he wants according to G =[ b ′–( b ′′′– M ′′′)] mod d . For arbitrary N , this process can be iterated in a straightforward manner. Full size image Clearly, this process can be repeated an arbitrary number of times, with Alice and Bob sharing 2 n –1 boxes for a task involving N =2 n dits. Note, however, that only n of these boxes are actively used in the protocol, in the sense that the outcome of the remaining ones is irrelevant for the correctness of the guess. Therefore, we now look at how the errors accumulate in the different stages of the nested protocol. The joint probability of success for two different boxes α and β is given by where the first term corresponds to both boxes succeeding, and the second term arises from error compensation: of the (d– 1) 2 “α wrong, β wrong′ events, only d –1 leads to a cancellation. We can now think of the probability of success for n +1 boxes as the joint success of n boxes and a single box: This recurrence can be solved for P s =[( d –1) E +]/] d , the probability of success of a noisy PR box, to finally obtain How to cite this article: Cavalcanti, D. et al . Macroscopically local correlations can violate information causality. Nat. Commun. 1:136 doi: 10.1038/ncomms1138 (2010).